Molecular mechanism of the assembly of an acid-sensing receptor ion channel complex Polycystic kidney disease (PKD) family proteins associate with transient receptor potential (TRP) channel family proteins to form functionally important complexes. PKD proteins differ from known ion channel-forming proteins and are generally thought to act as membrane receptors. Here we find that PKD1L3, a PKD protein, functions as a channel-forming subunit in an acid-sensing heteromeric complex formed by PKD1L3 and TRPP3, a TRP channel protein. Single amino-acid mutations in the putative pore region of both proteins alter the channel’s ion selectivity. The PKD1L3/TRPP3 complex in the plasma membrane of live cells contains one PKD1L3 and three TRPP3. A TRPP3 C-terminal coiled-coil domain forms a trimer in solution and in crystal, and has a crucial role in the assembly and surface expression of the PKD1L3/TRPP3 complex. These results demonstrate that PKD subunits constitute a new class of channel-forming proteins, enriching our understanding of the function of PKD proteins and PKD/TRPP complexes. Five human polycystic kidney disease (PKD) proteins are known to exist, with wide tissue distribution and limited knowledge of their biological functions [1] , [2] , [3] , [4] . Members of the PKD protein family associate with members of the transient receptor potential channel P subfamily (TRPP) to form heteromeric protein complexes. TRPP proteins belong to the large transient receptor potential (TRP) cation channel family that expresses in diverse species and cell types and has critical roles in sensory physiology [5] , [6] , [7] , [8] , [9] . The founding members of PKD and TRPP families, PKD1 (also known as polycystin-1) and TRPP2 (also known as polycystin-2 or PKD2), coassemble to form a receptor/ion channel complex [1] , [2] , [3] , [4] . Mutations in these proteins cause autosomal dominant PKD, one of the most common inherited human diseases [1] , [2] , [3] , [4] . PKD1L3, another PKD family member, interacts with another TRPP family member, TRPP3 (also known as polycystin-L or PKD2L1). These proteins colocalize in a subset of acid-sensing taste cells [10] , [11] , [12] , [13] ; these taste cells and HEK 293 cells heterologously expressing both proteins respond to extracellular acid [11] , [12] , [14] , [15] , [16] , making the PKD1L3/TRPP3 complex a good candidate for a sour taste receptor. Several lines of evidence from studies on animals and humans further support the hypothesis that the PKD1L3/TRPP3 complex is a candidate sour taste receptor. (i) Selective ablation of TRPP3-expressing taste cells abolishes all gustatory response to acidic stimuli [10] . (ii) Two patients with sour ageusia are reported to have no expression of TRPP3, PKD1L3 and several acid-sensing ion channel proteins in their taste cells [17] . (iii) TRPP3-expressing taste cells exhibit acid responses similar to those of exogenously expressed PKD1L3/TRPP3 complexes [12] . (iv) TRPP3 knockout mice show clear sour taste deficit [18] . Although no significant effect on sour taste was observed in PKD1L3 knockout mice [18] , [19] , and a proton current proposed to drive action potential firing in sour taste cells was unaffected by PKD1L3 knockout [20] , a role of PKD1L3 in sour taste could not be excluded because PKD1L3 function could have been compensated by other proteins in the knockout animals. PKD and TRPP proteins have markedly different molecular properties and functions. Human TRPP proteins have 613–968 amino acids and 6 transmembrane segments, with a pore-forming loop between the last two transmembrane segments, and they form ion channels [21] , [22] , [23] , [24] , [25] , [26] . PKD proteins, on the other hand, have 1,732–4,303 amino acids and 11 putative transmembrane segments, with a large (698–3,074 amino acids) extracellular N terminus containing well-recognized protein–protein, protein–saccharide and protein–ligand interaction motifs. PKD proteins are thus generally thought to function as cell surface receptors [1] , [2] , [3] , [4] . Intriguingly, the last six transmembrane segments of PKD proteins share significant amino-acid sequence homology with TRPP proteins [27] , and a putative pore region was suggested to be present in some PKD members, including PKD1L3 (ref. 28 ). If PKD proteins indeed function as channel-forming subunits, they would represent a novel family of ion channels. Although there is currently no experimental evidence demonstrating that PKD proteins are in fact channel-forming subunits, this possibility has been hinted. In a previous study on the PKD1/TRPP2 complex, we found that this complex contained three TRPP2 and one PKD1 when expressed in the plasma membrane of Xenopus oocytes [29] . As TRP channels are tetramers [6] , [8] , [9] , such a stoichiometry raises the possibility that PKD1 constitutes a pore-forming subunit in the PKD1/TRPP2 complex. However, this hypothesis could not be tested with PKD1 due to the lack of a reliable method to activate the PKD1/TRPP2 complex [29] . In this study, we take advantage of the fact that the PKD1L3/TRPP3 complex can be robustly activated by extracellular acid [11] , [12] , [14] , [15] , [16] and demonstrate that PKD1L3, a close relative of PKD1, is a channel-forming subunit. We also find that this complex contains one PKD1L3 and three TRPP3 subunits, and a TRPP3 C-terminal coiled-coil domain has a crucial role in determining this stoichiometry. PKD1L3 and TRPP3 form an acid-sensing ion channel With two-electrode voltage clamp (TEVC), we recorded robust acid-induced currents from Xenopus oocytes expressing PKD1L3 and TRPP3 ( Fig. 1a ). Currents were not detected when TRPP3 or PKD1L3 was expressed alone ( Fig. 1a ), or when TRPP3 or TRPP2 was coexpressed with PKD1 or PKD1L3, respectively ( Fig. 1b ). As reported in HEK 293T cells [14] , the PKD1L3/TRPP3 current was observed only when oocytes were neutralized after a brief low pH treatment (citric acid, pH 2.8), and this current was quickly and reversibly inhibited by reapplication of H + ( Fig. 1a ). This current could be an off-response [14] or could be due to the removal of proton blockage of open channels. As discussed in a previous study, such an off-response correlates well with the off-response associated with the perception of sour taste in mammals [14] . The current–voltage (I–V) relationship of the acid-induced current showed a reversal potential of −9.6±2.8 mV ( n =148) in a bath solution containing 100 mM NaCl ( Fig. 1c ), suggesting that the PKD1L3/TRPP3 channel has a similar permeability to Na + and K + . 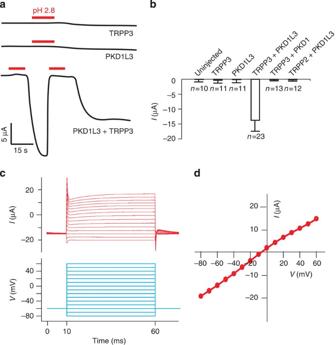Figure 1: The PKD1L3/TRPP3 complex functions as an acid-sensing ion channel. (a) Whole-cell current induced by citric acid (pH 2.8, red bar) in oocytes expressing the indicated subunit(s). Holding potential (HP)=−60 mV. (b) Bar graph comparing acid-induced currents in oocytes expressing the indicated subunit(s). HP=−80 mV. Results are shown as mean and s.d.n=number of oocytes. (c) Representative acid-induced whole-oocyte currents (upper panel) conducted by PKD1L3/TRPP3 channels under voltage clamp between −80 to +60 mV (lower panel). (d)I–Vcurve extracted fromc. Figure 1: The PKD1L3/TRPP3 complex functions as an acid-sensing ion channel. ( a ) Whole-cell current induced by citric acid (pH 2.8, red bar) in oocytes expressing the indicated subunit(s). Holding potential (HP)=−60 mV. ( b ) Bar graph comparing acid-induced currents in oocytes expressing the indicated subunit(s). HP=−80 mV. Results are shown as mean and s.d. n =number of oocytes. ( c ) Representative acid-induced whole-oocyte currents (upper panel) conducted by PKD1L3/TRPP3 channels under voltage clamp between −80 to +60 mV (lower panel). ( d ) I–V curve extracted from c . Full size image PKD1L3 is an ion channel pore-forming subunit We next investigated whether PKD1L3, as well as TRPP3, contribute to form the channel pore. A widely held and extensively tested prediction of channel-forming proteins is that mutating residues lining the ion conduction pathway significantly alters the ion selectivity (not simply current amplitude) of the channel. Based on amino-acid sequence alignment ( Fig. 2a ), a pore-forming loop has been proposed to exist between the last two transmembrane segments in both TRPP3 and PKD1L3 (ref. 28 ). To test whether these proteins are channel-forming subunits, we carried out extensive mutagenesis in this region of both proteins and examined the effect of the mutations on the ion selectivity of PKD1L3/TRPP3 channels. Dimethylamine + , trimethylamine + and Mg 2+ were chosen as charge carriers for their size and/or charge and compared to Na + . 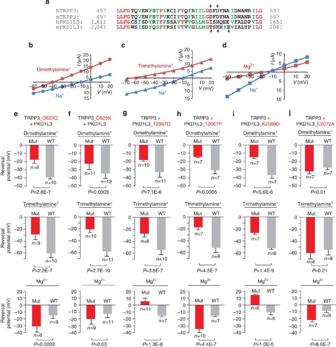Figure 2: Both PKD1L3 and TRPP3 line the pore. (a) Amino-acid sequence alignment of the putative pore region of human (h) and mouse (m) TRPP3 and PKD1L3. Red: identical; green: conserved. Residues marked by arrows were critical for ion selectivity. (b–d) RepresentativeI–Vcurves of acid-induced currents of WT PKD1L3/TRPP3 in a bath solution containing Na+, dimethylamine+, trimethylamine+or Mg2+. The two curves in each panel were obtained from the same oocyte. (e–j) Bar graph showing the reversal potential of currents recorded from WT (grey bars) or mutant (red bars) PKD1L3/TRPP3 complexes (mutation indicated at the top of each panel) in a bath solution containing dimethylamine+, trimethylamine+or Mg2+. All pairwise data were obtained from the same batch of oocytes and all pairwise comparisons are significantly different (P<0.05 as determined by unpaired two-tailed Student’st-test), except the middle panel inj. RepresentativeI–Vcurve for each condition is shown inSupplementary Fig. S2. Results are shown as mean and s.d.n=number of measurements. Figure 2b–d shows the I–V relationships of currents recorded from wild-type (WT) PKD1L3/TRPP3 channels in bath solutions containing 100 mM dimethylamine + , 100 mM trimethylamine + , 70 mM Mg 2+ or 100 mM Na + , with which each of the other ions was compared in the same oocyte. The reversal potential in dimethylamine + and trimethylamine + was −34.0±5.7 mV ( n =55) and −57.0±7.9 mV ( n =54), respectively ( Fig. 2b ), indicating that PKD1L3/TRPP3 channels are much less permeable to these ions than to Na + ( P Na : P dimethylamine : P trimethylamine =1:0.39:0.16 ). The reversal potential in Mg 2+ was −13.7±4.2 mV ( n =49), close to that in Na + ( Fig. 2d ), indicating that Mg 2+ permeates well through PKD1L3/TRPP3 channels ( P Na :P Mg =1:0.65). Figure 2: Both PKD1L3 and TRPP3 line the pore. ( a ) Amino-acid sequence alignment of the putative pore region of human (h) and mouse (m) TRPP3 and PKD1L3. Red: identical; green: conserved. Residues marked by arrows were critical for ion selectivity. ( b – d ) Representative I–V curves of acid-induced currents of WT PKD1L3/TRPP3 in a bath solution containing Na + , dimethylamine + , trimethylamine + or Mg 2+ . The two curves in each panel were obtained from the same oocyte. ( e – j ) Bar graph showing the reversal potential of currents recorded from WT (grey bars) or mutant (red bars) PKD1L3/TRPP3 complexes (mutation indicated at the top of each panel) in a bath solution containing dimethylamine + , trimethylamine + or Mg 2+ . All pairwise data were obtained from the same batch of oocytes and all pairwise comparisons are significantly different ( P <0.05 as determined by unpaired two-tailed Student’s t -test), except the middle panel in j . Representative I–V curve for each condition is shown in Supplementary Fig. S2 . Results are shown as mean and s.d. n =number of measurements. Full size image Our examination of the sequences suggested several residues that could line the pore in both TRPP3 and PKD1L3, including D523 and D525 in TRPP3 and T2067, K2069 and E2072 in PKD1L3. Mutations of these residues not only changed the amplitude of acid-induced currents in most cases ( Supplementary Fig. S1 ) but also changed the ion selectivity of PKD1L3/TRPP3 channels ( Fig. 2e–j , Table 1 , Supplementary Figs S2, S3 and Supplementary Table S1 ). For example, mutating D523 of TRPP3 to glutamine (D523Q) or D525 of TRPP3 to lysine (D525K) increased the relative permeability of dimethylamine + and trimethylamine + and decreased the relative permeability of Mg 2+ ( Fig. 2e , Table 1 and Supplementary Fig. S2a,b ). D523 of TRPP3 has also been shown to be important to Ca 2+ permeation of PKD1L3/TRPP3 channels [30] . When the two corresponding positions in PKD1L3, T2067 and K2069, were mutated to aspartic acid, all three ions became more permeant ( Fig. 2g , Table 1 and Supplementary Fig. S2c,e ). In both cases, the reversal potential of Mg 2+ even became positive ( Fig. 2g and Supplementary Fig. S2c,e ), indicating that Mg 2+ became more permeant than K + and Na + ( Table 1 ). In contrast, when T2067 was mutated to proline, the mutant channels became less permeable to Mg 2+ , albeit they still exhibited increased relative permeability to dimethylamine + and trimethylamine + ( Fig. 1h , Table 1 and Supplementary Fig. S2d ). The E2072A mutation slightly decreased the relative permeability of dimethylamine + but did not affect that of trimethylamine + ( Fig. 1j , Table 1 and Supplementary Fig. S2f ). However, it significantly decreased Mg 2+ permeability ( Fig. 1j , Table 1 and Supplementary Fig. S2f ). Table 1 Permeability ratios of WT PKD1L3/TRPP3 and the listed mutant channels for dimethylamine + , trimethylamine + and Mg 2+ . Full size table We also examined the relative permeability of WT channel and two mutant channels to N -methyl- D -glucamine (NMDG + ) and K + . NMDG + was only slightly permeant through WT channels, whereas K + was as permeant as Na + ( Supplementary Fig. S3 and Supplementary Table S1 ). The TRPP3_D523Q mutation altered the relative permeability of NMDG + ( Supplementary Fig. S3a and Supplementary Table S1 ), as it did for other ions ( Table 1 ). This mutation also affected K + permeation, as indicated by the more negative reversal potential in K + ( Supplementary Fig. S3a ). On the other hand, despite its strong effect on the relative permeability of dimethylamine + , trimethylamine + and Mg 2+ ( Table 1 ), the PKD1L3_K2069D mutation did not affect the relative permeability of NMDG + and K + ( Supplementary Fig. S3b and Supplementary Table S1 ). This is perhaps because the size of NMDG + and K + are either too big or too close to that of Na + such that their permeation is insensitive to this single mutation. Taken together, these results provide strong evidence that PKD1L3 and TRPP3 are both pore-forming subunits. The TRPP3 homomeric complex contains three TRPP3 subunits TRP channels are tetramers [6] , [8] , [9] . We previously showed that the PKD1/TRPP2 complex expressed in the oocyte plasma membrane contains one PKD1 and three TRPP2. (ref. 29 ) What is the subunit stoichiometry of heteromeric PKD1L3/TRPP3 channels? To address this question, we used a single-molecule photobleaching method that allows subunit counting of membrane proteins in live cells [31] . In this approach, enhanced green fluorescent protein (EGFP)-tagged proteins are expressed in the plasma membrane of Xenopus oocytes at low levels and visualized with total internal reflection fluorescence (TIRF) microscopy. EGFP bleaches with continuous excitation. The number of EGFP bleaching steps represents the number of tagged subunits in a complex. When PKD1L3–EGFP was expressed alone, few EGFP spots were seen on the oocyte surface ( Supplementary Fig. S4 ), suggesting that coexpression of TRPP3 is required to bring PKD1L3 to the surface. On the other hand, when TRPP3–EGFP was expressed alone, numerous fluorescent spots were seen on the plasma membrane ( Fig. 3a ), indicating that TRPP3 can reach the surface membrane either on its own or, possibly, in complex with an unknown endogenous oocyte protein. Regardless, the TRPP3 complex that lacks PKD1L3 does not respond to acid ( Fig. 1a ). Green fluorescence spots observed with TIRF that are immobile were selected for further analysis, each spot representing a single TRPP3 homomeric complex ( Fig. 3a , green circles). In the photobleaching experiments, most selected spots showed 1, 2 or 3 EGFP bleaching steps, whereas a small number of spots bleached in 4 steps ( Fig. 3b ). The distribution of 1-to-3 bleaching steps was well fit by a binomial distribution, in which each spot contains three EGFP molecules and the probability of EGFP being fluorescent is 70% ( Fig. 3c ), a probability of EGFP fluorescence similar to what has been seen in fusions to other ion channels [29] , [31] , [32] . The presence of the small number of four EGFP bleaching spots could be due to occasional colocalization of two complexes. The distribution of EGFP bleaching steps was poorly fit by a binomial distribution that assumes four EGFPs in one spot ( Supplementary Fig. S5a ). This result indicates that the TRPP3 homomeric complex in the plasma membrane of live oocytes contains three TRPP3 subunits. 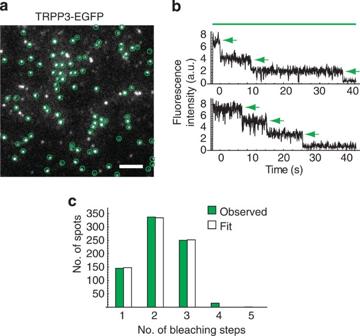Figure 3: Homomeric TRPP3 complexes on the plasma membrane ofXenopusoocytes contain three TRPP3 subunits. (a) TIRF image from an oocyte expressing TRPP3–EGFP. Immobile spots were selected (circles) for photobleaching analysis. Scale bar, 2 μm. (b) Time course of photobleaching of two representative spots ina, showing three EGFP bleaching steps (arrows). Green bar indicates EGFP excitation. (c) Distribution of observed and calculated bleaching steps for TRPP3–EGFP fluorescence spots. The 1–3 step distribution (green bars) is well fit by a binomial distribution (white bars) that assumes that each spot contains three EGFPs and that the probability of EGFP to be fluorescent is 70%. Figure 3: Homomeric TRPP3 complexes on the plasma membrane of Xenopus oocytes contain three TRPP3 subunits. ( a ) TIRF image from an oocyte expressing TRPP3–EGFP. Immobile spots were selected (circles) for photobleaching analysis. Scale bar, 2 μm. ( b ) Time course of photobleaching of two representative spots in a , showing three EGFP bleaching steps (arrows). Green bar indicates EGFP excitation. ( c ) Distribution of observed and calculated bleaching steps for TRPP3–EGFP fluorescence spots. The 1–3 step distribution (green bars) is well fit by a binomial distribution (white bars) that assumes that each spot contains three EGFPs and that the probability of EGFP to be fluorescent is 70%. Full size image The PKD1L3/TRPP3 complex contains one PKD1L3 and three TRPP3 To determine the subunit stoichiometry of the PKD1L3/TRPP3 complex, we coexpressed EGFP-tagged TRPP3 with mCherry-tagged PKD1L3. Under these conditions, we observed numerous red fluorescent spots on the cell surface ( Fig. 4a ), supporting the notion that coexpression with TRPP3 helps transport PKD1L3 to the plasma membrane. Fluorescent spots showing green and red dual fluorescence, which are expected to be PKD1L3/TRPP3 complexes, were selected for further analysis. Again, most spots that had both green and red fluorescence showed 1, 2 or 3 EGFP bleaching steps, while a small number of spots bleached in 4 steps ( Fig. 4b ). The distribution of 1-to-3 bleaching steps was well fit by a binomial distribution, in which each spot contains three EGFP molecules and the probability of EGFP being fluorescent is 78% ( Fig. 4c ). The distribution of EGFP bleaching steps was poorly fit by a binomial distribution that assumes four EGFPs in one spot ( Supplementary Fig. S5b ). Because mCherry photobleaches too quickly to count bleaching steps, we switched the tags on TRPP3 and PKD1L3 and coexpressed TRPP3–mCherry with PKD1L3–EGFP ( Fig. 4d ). Now almost all spots that had both green and red fluorescence showed only one EGFP bleaching step ( Fig. 4e ). Both the TRPP3–EGFP/PKD1L3–mCherry complex and the TRPP3–mCherry/PKD1L3–EGFP complex generated acid-induced currents when expressed at high levels ( Supplementary Fig. S6 ). Taken together, the results indicate that the functional PKD1L3/TRPP3 complex in the plasma membrane of live oocytes contains one PKD1L3 and three TRPP3 subunits ( Fig. 4g ), conforming to the tetrameric quaternary structure of TRP channels and consistent with PKD1L3 being a channel-forming subunit. 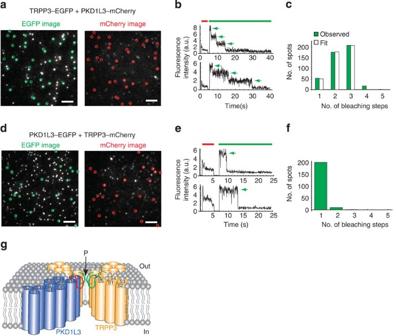Figure 4: The PKD1L3/TRPP3 heteromeric channel has a 1:3 subunit stoichiometry. (a,d) TIRF images of EGFP fluorescence from an oocyte expressing the indicated constructs, showing spots that exhibited EGFP and mCherry dual fluorescence and were immobile (circles). Other spots do not fit analysis criteria. Scale bar, 2 μm. (b,e) Time course of photobleaching of two representative dual-fluorescence spots of either TRPP3–EGFP+PKD1L3–mCherry (b) or PKD1L3–EGFP+TRPP3–mCherry (e), showing EGFP bleaching steps (arrows). EGFP and mCherry excitation is indicated by green and red bar, respectively. (c,f) Distribution of observed EGFP bleaching steps (green bars) for dual-fluorescence spots of either TRPP3–EGFP+PKD1L3–mCherry (c) or PKD1L3–EGFP+TRPP3–mCherry (f). Inc, observed EGFP bleaching steps are compared to a binomial distribution assuming that three EGFP molecules exist in each spot and based on 78% of EGFPs being fluorescent (white bars). (g) Schematic diagram of the heteromeric PKD1L3/TRPP3 channel viewed from the side. P: channel pore. Green and red loops depict the putative selectivity filter formed by the pore loops shown inFig. 2a. The inner pore is presumed to be lined by the 11th transmembrane segment (S11) of PKD1L3 and the 6th transmembrane segment (S6) of TRPP3. Figure 4: The PKD1L3/TRPP3 heteromeric channel has a 1:3 subunit stoichiometry. ( a , d ) TIRF images of EGFP fluorescence from an oocyte expressing the indicated constructs, showing spots that exhibited EGFP and mCherry dual fluorescence and were immobile (circles). Other spots do not fit analysis criteria. Scale bar, 2 μm. ( b , e ) Time course of photobleaching of two representative dual-fluorescence spots of either TRPP3–EGFP+PKD1L3–mCherry ( b ) or PKD1L3–EGFP+TRPP3–mCherry ( e ), showing EGFP bleaching steps (arrows). EGFP and mCherry excitation is indicated by green and red bar, respectively. ( c , f ) Distribution of observed EGFP bleaching steps (green bars) for dual-fluorescence spots of either TRPP3–EGFP+PKD1L3–mCherry ( c ) or PKD1L3–EGFP+TRPP3–mCherry ( f ). In c , observed EGFP bleaching steps are compared to a binomial distribution assuming that three EGFP molecules exist in each spot and based on 78% of EGFPs being fluorescent (white bars). ( g ) Schematic diagram of the heteromeric PKD1L3/TRPP3 channel viewed from the side. P: channel pore. Green and red loops depict the putative selectivity filter formed by the pore loops shown in Fig. 2a . The inner pore is presumed to be lined by the 11th transmembrane segment (S11) of PKD1L3 and the 6th transmembrane segment (S6) of TRPP3. Full size image TRPP3 C-terminus trimerizes through a coiled-coil domain Previously, we showed that a C-terminal coiled-coil domain of TRPP2 forms a trimer and has a crucial role in the assembly of TRPP2 homomeric trimers and TRPP2/PKD1 heteromeric complexes [29] . We aligned TRPP2 and TRPP3 C-termini and found a putative coiled-coil domain in TRPP3 ( Fig. 5a ; also see ref. 33 ). All hydrophobic amino acids important for the TRPP2 coiled-coil interaction [29] are conserved in TRPP3 ( Fig. 5b ). We solved the crystal structure of a TRPP3 C-terminal fragment (G699–W743) containing the coiled-coil domain to 2.8 Å resolution ( Fig. 5c , Supplementary Table S2 and Supplementary Fig. S7 ) and found it to form a trimer similar to that of the TRPP2 coiled-coil domain ( Fig. 5e ). The TRPP3 coiled-coil trimer structure reported here is virtually identical to a recently released crystal structure of a similar TRPP3 region [34] . 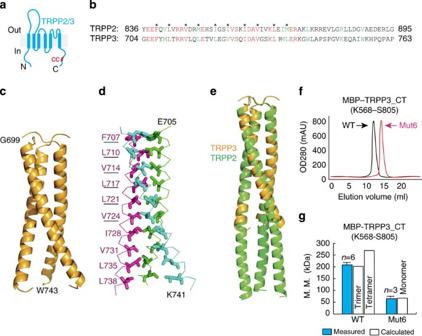Figure 5: The TRPP3 C-terminus forms a trimer. (a) Putative transmembrane topology of TRPP2 and TRPP3. The C terminus of both proteins contains a coiled-coil domain (red bar). (b) Amino-acid sequence alignment of TRPP2 and TRPP3 coiled-coil domains. Red: identical; green: conserved. Asterisks indicate hydrophobic residues at the 1st and 4th positions in characteristic heptad repeats of canonical coiled-coil domains. (c) Crystal structure of TRPP3–G699–W743 fragment, showing that the TRPP3 coiled-coil domain forms a trimer. (d) Side chains, shown in sticks, of hydrophobic residues involved in the formation of the coiled-coil domain trimer. The underlined amino acids were mutated to alanine to generate mut6. (e) Superposition of the structures of TRPP3 and TRPP2 coiled-coil domains (PDB: 3HRN). (f) Gel filtration profile of MBP-tagged WT TRPP3 C-terminal fragment (TRPP3_CT) and TRPP3_CT_mut6. The right shift of the latter indicates a decrease in molecular mass. (g) Bar graph comparing the calculated and measured molecular masses of MBP–TRPP3_CT and MBP–TRPP3_CT_mut6. Measured molecular masses were obtained by static light scattering. Calculated molecular masses were obtained assuming that the protein is a monomer (for mut6), a trimer (for WT) or a tetramer (for WT). Figure 5: The TRPP3 C-terminus forms a trimer. ( a ) Putative transmembrane topology of TRPP2 and TRPP3. The C terminus of both proteins contains a coiled-coil domain (red bar). ( b ) Amino-acid sequence alignment of TRPP2 and TRPP3 coiled-coil domains. Red: identical; green: conserved. Asterisks indicate hydrophobic residues at the 1st and 4th positions in characteristic heptad repeats of canonical coiled-coil domains. ( c ) Crystal structure of TRPP3–G699–W743 fragment, showing that the TRPP3 coiled-coil domain forms a trimer. ( d ) Side chains, shown in sticks, of hydrophobic residues involved in the formation of the coiled-coil domain trimer. The underlined amino acids were mutated to alanine to generate mut6. ( e ) Superposition of the structures of TRPP3 and TRPP2 coiled-coil domains (PDB: 3HRN). ( f ) Gel filtration profile of MBP-tagged WT TRPP3 C-terminal fragment (TRPP3_CT) and TRPP3_CT_mut6. The right shift of the latter indicates a decrease in molecular mass. ( g ) Bar graph comparing the calculated and measured molecular masses of MBP–TRPP3_CT and MBP–TRPP3_CT_mut6. Measured molecular masses were obtained by static light scattering. Calculated molecular masses were obtained assuming that the protein is a monomer (for mut6), a trimer (for WT) or a tetramer (for WT). Full size image To evaluate the importance of the coiled-coil domain trimer in the assembly of TRPP3 homomeric complexes and PKD1L3/TRPP3 heteromeric complexes, we simultaneously replaced six hydrophobic amino acids involved in the coiled-coil interaction to alanine ( Fig. 5d ), creating a mutation called mut6. This mutation disrupted the association of TRPP3 C terminus, as revealed by gel filtration chromatography ( Fig. 5f ) and static light scattering ( Fig. 5g ) of a maltose-binding protein (MBP)-tagged C-terminal protein (MBP–TRPP3_CT, amino acids K568–S805). Gel filtration showed a right shift of mut6 MBP–TRPP3_CT in comparison with WT MBP–TRPP3_CT, indicating a decrease of the molecular mass of the MBP–TRPP3_CT complex ( Fig. 5f ). The molecular mass determined by light scattering showed that WT MBP–TRPP3_CT formed a trimer in solution ( Fig. 5g ), consistent with the crystal structure ( Fig. 5c ) and a previous report [33] , but that mut6 MBP–TRPP3_CT was a monomer ( Fig. 5g ). These results indicate that the coiled-coil domain has a critical role in the trimeric assembly of TRPP3 C terminus. Coiled-coil trimer is critical for TRPP3 homomeric assembly To test the effect of the TRPP3 coiled-coil trimer interaction on the assembly of the full-length TRPP3 homomeric complex, two TRPP3 mutants were made to disrupt the coiled-coil trimer: one was TRPP3 with mut6 (named TRPP3_mut6) and the other was TRPP3 with its coiled-coil domain (G704-K741) replaced with eight glycines (named TRPP3_CCto8G). FLAG-tagged TRPP3 carrying each mutation was coexpressed with HA-tagged WT TRPP3 in Xenopus oocytes. Coimmunoprecipitation showed that homomeric TRPP3 association was markedly weakened by both mutations ( Fig. 6a ). TIRF imaging further showed that mut6 greatly decreased the surface expression of TRPP3 homomeric complexes in oocytes ( Fig. 6b ). These results indicate that the integrity of the TRPP3 C-terminal trimer is critical for the assembly of the homomeric TRPP3 complex and its surface expression. 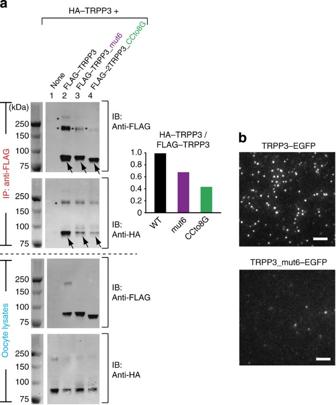Figure 6: The TRPP3 coiled-coil domain trimer is important for the assembly and surface expression of homomeric TRPP3 complexes. (a) HA- and FLAG-tagged full-length TRPP3, as indicated on top, were expressed inXenopusoocytes and immunoprecipitated (IP) with anti-FLAG antibody coated beads. All proteins had comparable expression as can be seen from the lysate samples (lower two gels). Reduced amount of HA-tagged TRPP3 was co-IPed with FLAG-tagged TRPP3 mutants that lack the coiled-coil trimer interaction (upper gel, lanes 3 and 4). IB: immunoblot. On SDS–polyacrylamide gel electrophoresis, WT TRPP3 gave rise to a monomeric band at ~90 kDa (arrows) and two oligomeric bands with molecular masses of ~200 and >250 kDa (asterisks). The oligomeric complexes appeared even at more severe denaturing and reducing conditions (Supplementary Fig. S8). The two FLAG-tagged TRPP3 mutants showed reduced amount of both oligomeric bands, suggesting a weakened homomeric assembly of TRPP3 (upper gel immunobloted with anti-Flag antibody, lanes 3 and 4; also seeFig. 7c,d). Bar graph at right shows the normalized ratio of the intensity of HA–TRPP3 (WT or mutants as indicated at bottom)/Flag–TRPP3. The sum of the intensity of all monomeric and oligomeric bands for each TRPP3 protein was used in the calculation. A smaller ratio suggests a weakened association between HA–TRPP3 and Flag–TRPP3. (b) TIRF images of EGFP fluorescence from oocytes expressing the indicated constructs. Upper panel was a duplication ofFigure 3a. Scale bar, 2 μm. Figure 6: The TRPP3 coiled-coil domain trimer is important for the assembly and surface expression of homomeric TRPP3 complexes. ( a ) HA- and FLAG-tagged full-length TRPP3, as indicated on top, were expressed in Xenopus oocytes and immunoprecipitated (IP) with anti-FLAG antibody coated beads. All proteins had comparable expression as can be seen from the lysate samples (lower two gels). Reduced amount of HA-tagged TRPP3 was co-IPed with FLAG-tagged TRPP3 mutants that lack the coiled-coil trimer interaction (upper gel, lanes 3 and 4). IB: immunoblot. On SDS–polyacrylamide gel electrophoresis, WT TRPP3 gave rise to a monomeric band at ~90 kDa (arrows) and two oligomeric bands with molecular masses of ~200 and >250 kDa (asterisks). The oligomeric complexes appeared even at more severe denaturing and reducing conditions ( Supplementary Fig. S8 ). The two FLAG-tagged TRPP3 mutants showed reduced amount of both oligomeric bands, suggesting a weakened homomeric assembly of TRPP3 (upper gel immunobloted with anti-Flag antibody, lanes 3 and 4; also see Fig. 7c,d ). Bar graph at right shows the normalized ratio of the intensity of HA–TRPP3 (WT or mutants as indicated at bottom)/Flag–TRPP3. The sum of the intensity of all monomeric and oligomeric bands for each TRPP3 protein was used in the calculation. A smaller ratio suggests a weakened association between HA–TRPP3 and Flag–TRPP3. ( b ) TIRF images of EGFP fluorescence from oocytes expressing the indicated constructs. Upper panel was a duplication of Figure 3a . Scale bar, 2 μm. Full size image TRPP3 trimer is crucial for PKD1L3/TRPP3 surface expression When PKD1L3 was coexpressed in oocytes with either TRPP3_mut6 or TRPP3_CCto8G, acid-induced currents were greatly diminished ( Fig. 7a ). This loss of current was primarily due to a diminished surface expression of the mutant PKD1L3/TRPP3 complexes. TIRF imaging showed that mut6 greatly decreased the surface expression of PKD1L3/TRPP3 complexes in oocytes ( Fig. 7b ). This result was confirmed by detecting surface protein with surface biotinylation ( Fig. 7c ). While FLAG-tagged WT TRPP3 (FLAG–TRPP3) showed detectable expression on the plasma membrane ( Fig. 7c , lanes 2 in upper gels), FLAG–TRPP3_mut6 showed little surface expression ( Fig. 7c , lane 5). Likewise, while coexpressing WT PKD1L3 and WT TRPP3 produced measurable surface expression of both proteins ( Fig. 7c , lane 4), coexpressing WT PKD1L3 with either of the two aforementioned TRPP3 mutants produced greatly reduced surface expression of either protein ( Fig. 7c , lanes 6 and 7 and bar graph). Consistent with TIRF imaging of PKD1L3 alone ( Supplementary Fig. S4 ), surface biotinylation showed that PKD1L3 expressed poorly on the plasma membrane on its own ( Fig. 7c , lane 3). These results indicate that the TRPP3 coiled-coil trimer is crucial for the assembly and surface expression of PKD1L3/TRPP3 complexes. 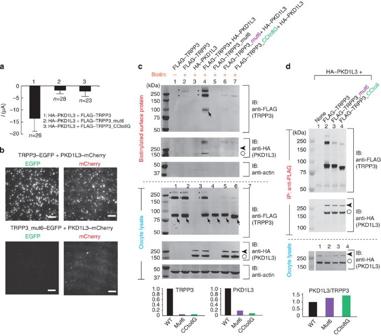Figure 7: The TRPP3 coiled-coil domain trimer is essential for the surface expression of the PKD1L3/TRPP3 complex. (a) Bar graph comparing acid-induced whole-cell currents from oocytes expressing the indicated constructs. (b) TIRF images of both EGFP and mCherry fluorescence from oocytes expressing the indicated constructs. The images for both combinations were obtained from oocytes injected with the same amount of cRNAs and on the same day after injection, and are representative of >6 different oocytes. Scale bar, 2 μm. (c) Western blot following SDS–polyacrylamide gel electrophoresis (PAGE) showing TRPP3 and PKD1L3 expressed on the plasma membrane (upper gels) and in the lysate (lower gels) of oocytes expressing the indicated constructs. The actin control shows that only surface proteins were biotinylated. Monomeric and oligomeric TRPP3 are indicated by arrows and asterisks. PKD1L3 showed a full-length band (>250 kDa, arrowheads) and a cleaved band (~180 kDa, open circles; lower gel, lanes 3, 4, 6 and 7). Disruption of the TRPP3 coiled-coil domain trimer reduced the surface expression of TRPP3 (upper gel, lanes 5–7) and PKD1L3 (upper gel, lanes 6 and 7). Bar graphs at the bottom show the normalized intensity of surface TRPP3 or PKD1L3 proteins when PKD1L3 was coexpressed with WT or the indicated mutant TRPP3. Data were obtained from lines 4, 6 and 7 on the top two gels. The sum of the intensity of all monomeric and oligomeric bands for each protein was used in the calculation. (d) Western blot following SDS–PAGE showing that PKD1L3 (HA-tagged) can be coimmunoprecipitated with all indicated TRPP3 constructs (FLAG-tagged). Monomeric and oligomeric TRPP3 are indicated by arrows and asterisks. Full-length and cleaved PKD1L3 are indicated by arrowheads and open circles. Bar graph at the bottom shows the normalized ratio of the intensity of HA–PKD1L3/FLAG–TRPP3 (WT or the indicated mutants). Figure 7: The TRPP3 coiled-coil domain trimer is essential for the surface expression of the PKD1L3/TRPP3 complex. ( a ) Bar graph comparing acid-induced whole-cell currents from oocytes expressing the indicated constructs. ( b ) TIRF images of both EGFP and mCherry fluorescence from oocytes expressing the indicated constructs. The images for both combinations were obtained from oocytes injected with the same amount of cRNAs and on the same day after injection, and are representative of >6 different oocytes. Scale bar, 2 μm. ( c ) Western blot following SDS–polyacrylamide gel electrophoresis (PAGE) showing TRPP3 and PKD1L3 expressed on the plasma membrane (upper gels) and in the lysate (lower gels) of oocytes expressing the indicated constructs. The actin control shows that only surface proteins were biotinylated. Monomeric and oligomeric TRPP3 are indicated by arrows and asterisks. PKD1L3 showed a full-length band (>250 kDa, arrowheads) and a cleaved band (~180 kDa, open circles; lower gel, lanes 3, 4, 6 and 7). Disruption of the TRPP3 coiled-coil domain trimer reduced the surface expression of TRPP3 (upper gel, lanes 5–7) and PKD1L3 (upper gel, lanes 6 and 7). Bar graphs at the bottom show the normalized intensity of surface TRPP3 or PKD1L3 proteins when PKD1L3 was coexpressed with WT or the indicated mutant TRPP3. Data were obtained from lines 4, 6 and 7 on the top two gels. The sum of the intensity of all monomeric and oligomeric bands for each protein was used in the calculation. ( d ) Western blot following SDS–PAGE showing that PKD1L3 (HA-tagged) can be coimmunoprecipitated with all indicated TRPP3 constructs (FLAG-tagged). Monomeric and oligomeric TRPP3 are indicated by arrows and asterisks. Full-length and cleaved PKD1L3 are indicated by arrowheads and open circles. Bar graph at the bottom shows the normalized ratio of the intensity of HA–PKD1L3/FLAG–TRPP3 (WT or the indicated mutants). Full size image Although the above TRPP3 coiled-coil mutations attenuated the surface expression of the PKD1L3/TRPP3 complex, they did not disrupt the association between PKD1L3 and TRPP3 ( Fig. 7d ). When HA–PKD1L3 was coexpressed with FLAG–TRPP3, FLAG–TRPP3_mut6 or FLAG–TRPP3_CCto8G in oocytes, it could be coimmunoprecipitated by an anti-FLAG antibody in all three cases ( Fig. 7d , lanes 2–4 and bar graph). This observation is consistent with a previous study reporting that PKD1L3 and TRPP3 can associate through their transmembrane segments [35] . Taken together, these results indicate that although the TRPP3 coiled-coil domain is not necessary for the association between TRPP3 and PKD1L3, it is essential for the trafficking of the PKD1L3/TRPP3 complex to the plasma membrane. One possible explanation for this dichotomy is that the complex assembled between PKD1L3 and TRPP3 without the C-terminal coiled-coil trimer has an incorrect subunit stoichiometry and cannot pass oocyte’s quality-control machinery. Mutations of residues that line the ion conduction pathway of an ion channel usually significantly alter its ion selectivity. This concept has often been applied to test whether a protein is an ion channel-forming subunit [36] , [37] , [38] . On the other hand, mutations of non-pore lining regulatory proteins that even interact directly with ion channels rarely affect the channels’ ion selectivity. To our knowledge, the only reported non-pore lining protein whose mutations affect a channel’s ion selectivity is mink (KCNE1), a K + channel regulatory subunit. In that case, however, only one residue was found that, when mutated, was able to increase the relative permeability of one ion (Na + ) by sevenfold (ref. 39 ). In this study, we found that single amino-acid mutations at three positions in PKD1L3 greatly changed the permeability of the PKD1L3/TRPP3 complex to three different cations ( Fig. 2 , Table 1 and Supplementary Fig. S2 ). These results strongly support the notion that PKD1L3 regulates the TRPP3 channel directly by coassembling with it to form the channel pore, showing that a member of the PKD family functions as a channel-forming subunit in addition to its possible role as a cell surface receptor. Whether other PKD proteins also function as channel-forming subunits remains to be determined. It is interesting to note that although PKD1 has been postulated to function solely as a regulator of the TRPP2 channel [1] , [40] , a putative pore-lining region also exists in PKD1 and the PKD1/TRPP2 complex also has a 1:3 stoichiometry [29] . It is possible that PKD protein serving as a pore-forming subunit may be a common feature of PKD/TRPP complexes. The TRPP2 coiled-coil domain forms a trimer and mediate the homomeric trimer assembly of the TRPP2 C terminus [29] , [33] , [41] and of full-length TRPP2 [29] . In this study we found that a similar coiled-coil domain is present in TRPP3, forms a trimer, and is critical for the trimeric assembly of the TRPP3 C terminus and of full-length TRPP3. Amino-acid sequence alignment suggests that a coiled-coil domain also exists in the C terminus of TRPP5 (also known as polycystin-L2 or PKD2L2), the third TRPP family protein [42] . This conservation suggests that homomeric trimer assembly may be a common property of the TRPP subfamily. A possible utility of forming a stable homotrimer rather than a stable homotetramer is that it allows the TRPP trimer to associate with either a fourth TRPP subunit to form a homomeric complex [43] or other channel-forming subunits like PKD proteins to form a hetromeric complex. A similar heteromeric assembly mechanism is seen in the cyclic nucleotide-gated channels of rod photoreceptors. This channel contains three A1 and one B1 subunits, and that this 3:1 stoichiometry is determined by a trimer-forming coiled-coil domain in the C terminus of the A1 subunit [44] . The C-terminal coiled-coil domain is critical for the direct interaction between TRPP2 and PKD1 and the assembly of the TRPP2/PKD1 complex [29] , [45] , [46] . The molecular determinants of TRPP3 and PKD1L3 association remain to be determined. The transmembrane domains have been reported to be important [35] . Disruption of the TRPP3 coiled-coil trimer does not eliminate direct association of TRPP3 and PKD1L3 ( Fig. 7d ), but it greatly reduces the surface expression of the PKD1L3/TRPP3 complex ( Figs 7b ). Thus, the C-terminal coiled-coil domain is essential for the proper assembly of both TRPP2/PKD1 and PKD1L3/TRPP3 complexes. In conclusion, we find that PKD1L3 functions as a channel-forming subunit and associates with TRPP3 in a 1:3 stoichiometry to form an acid-activated heteromeric channel. As a candidate sour taste receptor, PKD1L3 and TRPP3 colocalize in sour taste cells [10] , [11] , [12] , [13] . Besides, both TRPP3 and PKD1L3 are widely expressed and their expression overlaps in many tissues [28] , [47] , suggesting that the PKD1L3/TRPP3 complex may exist in tissues other than the tongue. The physiological role of PKD1L3/TRPP3 complexes in those tissues remains to be explored. Constructs and cloning Human TRPP3 (NCBI accession number NM_016112) and mouse PKD1L3 (AY164486) were used. The construct for HA-tagged PKD1L3 was described previously [6] . All mutations were checked by sequencing. TRPP3 constructs used for protein purification for light scattering experiments were cloned into a modified pCDFduet-1 vector (Novagen) containing an N-terminal MBP complementary DNA (cDNA). The TRPP3 C terminus construct used for crystallization was cloned into the pCDFduet-1 vector (Novagen). For constructs used for in vitro RNA synthesis, cDNAs were cloned into a modified pGEMHE vector. Constructs used in TIRF imaging experiments were cloned into a modified pGEMHE vector containing the cDNA for EGFP or mCherry. A flexible linker (SRGTSGGSGGSRGSGGSGG) was added between the fluorescent proteins and our constructs. Electrophysiology cRNA (antisense RNA) was synthesized in vitro and injected into Xenopus oocytes at 15 ng per oocyte. The injected RNA has a molar ratio of TRPP3:PKD1L3=1:3 to ensure an excess amount of PKD1L3. Whole-oocyte currents were recorded from oocytes 4 to 5 days after injection using TEVC. Solutions Standard bath solution contains 100 mM NaCl, 0.5 mM MgCl 2 and 2 mM HEPES (pH 7.5). pH was adjusted with NaOH. Acid solution was generated by adding citric acid into the bath solution until pH reached 2.8. For solutions used in the ion permeability assay, 100 mM NaCl in the standard solution was replaced with 100 mM dimethylamine hydrochloride, 100 mM trimethylamine hydrochloride, 70 mM MgCl 2 , 100 mM NMDG hydrochloride or 100 mM KCl. pH was adjusted to 7.5 with dimethylamine, trimethylamine or NMDG, respectively. Protocols For TEVC experiments, oocytes were held at −60 or −80 mV. Acid solution was applied for 12 s (flow speed is ~1.5 ml min −1 ) then washed away with bath solution. To measure current–voltage ( I – V ) relationships, 50-ms voltage steps from −80 to +60 mV were applied in 10-mV increments. For reversal potential measurements, the I – V protocol was alternated with voltage ramps from −70 to +60 mV in 160 ms. During the experiment, oocytes were first kept in the standard bath solution and voltage steps were applied to monitor the leak current (oocytes with leak currents bigger than 0.5 μA at −80 mV were discarded). Acid solution was applied to qualified oocytes for 12 s followed by washing with the solution containing dimethylamine + , trimethylamine + or Mg 2+ until the current reached its peak amplitude (monitored with voltage ramps). Subsequently, the I–V protocol was reapplied for extracting I–V curves and the reversal potential for the test ion. Oocytes were then washed with the standard solution while monitoring with voltage ramps until the reversal potential shift stopped. Finally, another voltage step protocol was applied for extracting the I–V curve and reversal potential in Na + . Relative permeabilities for monovalent cations were calculated based on changes of reversal potential upon switching the bath solution of NaCl to the test solutions. The permeability ratios, P x/ P Na , were calculated according to the equation derived from the Goldmann-Hodgkin-Katz (GHK) equation, [48] where E rev is the reversal potential, Δ E rev =E rev,X − E rev,Na , F is Faraday’s constant, R is the universal gas constant, and T is the absolute temperature. We considered the effect of Mg 2+ in the monovalent cation solutions negligible. P Mg / P Na was calculated from the change of reversal potential when Na + was replaced by Mg 2+ in the bath solution using the equation Activity coefficients for NaCl and MgCl 2 were determined from the tables of Robinson and Stokes [49] , and those for dimethylamine + and trimethylamine + were assumed to be equal to that of Na + . Data were presented as mean±s.d. Statistical significance was determined by unpaired two-tailed Student’s t -test. TIRF microscopy and EGFP bleaching steps The detailed methods have been described previously [29] , [31] . Oocytes were used at 24–48 h after cRNA injection. mCherry and EGFP fluorescence was recorded as movie and fluorescent spots that were immobile during the movie were selected and the number of EGFP bleaching steps was manually counted. Protein fragment expression and purification The TRPP3 C-terminal fragment (His6–TRPP3_K568-S805) used for crystallization was expressed in Rosetta (DE3) cells (Novagen). Bacteria were lysed with a Branson digital sonifier in a lysis solution containing 50 mM Tris–HCl, 250 mM NaCl, 2.5% glycerol, and 7 mM β-mercaptoethanol (pH 7.8). Protein was pulled downed with Ni-NTA His·Bind beads (Novagen) and eluted from the beads with 250 mM imidazole. The His 6 tag was removed by incubating overnight with thrombin (Sigma) at 20 °C. The protein was then purified with a Superose 12 column (GE Healthcare) on a Amersham Pharmacia ÄKTA Purifier in a solution contained 250 mM NaCl, 1% glycerol, 10 mM HEPES, pH 7.5. The TRPP3 C-terminal fragment used for light scattering was expressed as an MBP-tagged protein, purified with an amylose resin (New England Biolabs), and eluted from the beads with 20 mM maltose. The protein was then purified with a Superose 6 column (GE Healthcare). Detailed methods for protein purification have been described previously [29] . Light scattering measurements Purified protein samples were concentrated to 10 mg ml −1 . Protein (50 μl) was loaded on a gel filtration column Protein KW-804 (Shodex) with a solution containing 200 mM NaCl and 100 mM Tris–HCl (pH 7.5). Eluates were examined by static light-scattering (Wyatt Technology). Structure determination Crystallization of TRPP3_K568-S805 was carried out with the hanging-drop vapour diffusion method at 20 °C. The protein concentration was 20 mg ml −1 and the reservoir solution contained 18–20% PEG 8000, 100 mM HEPES, pH 7.5. Drops were set up with 1.6 μl protein+0.4 μl 39 mM HEGA-9 (additive)+2 μl reservoir solution. Crystals were rinsed in Paratone-N (Hampton Research) and flash-frozen in liquid nitrogen for data collection at 100 K. X-ray diffraction data were collected at the National Synchrotron Light Source beamline X4C on a Mar CCD ( λ =0.979 Å). The diffraction images were processed and scaled with the HKL package [50] . The crystal belongs to space group P321 with cell dimensions a = b =44.5 Å, c =62.3 Å, α = β =90°, γ =120°. The asymmetric unit was too small for the trimer of TRPP3_K568-S805 fragment, suggesting that the protein underwent unintended proteolysis during crystallization. The TRPP2 coiled-coil domain structure (PDB code 3HRO) was tried as the search model for molecular replacement in PHASER [51] and the replacement solution was found. The atomic model of the TRPP3 coiled-coil domain was built into the electron density maps using COOT [52] . Structure refinement was carried out with Crystallography & NMR system (CNS) [53] . The final model has an R -factor of 23.5% and an R free value of 28.6%, with 100% of the residues within the most favoured regions of the Ramachandran plot. Only the G699–W743 region was seen in the final crystal structure. Data collection and refinement statistics are summarized in Supplementary Table S2 , and a sample electron density map is shown in Supplementary Fig. S7 . All structural graphics were prepared using PyMOL (The PyMol Molecular Graphics System). Coimmunoprecipitation Xenopus Oocytes were injected with 15 ng per oocyte cRNA and incubated at 18 °C for 4 days before use. Twenty oocytes were used for each RNA combination. Oocytes were washed with cold 1 × PBS for three times and kept in a lysis solution containing 1 × PBS, 1 mM EDTA, 10% glycerol, 1% n - D odecyl β- D -maltoside (DDM) and 1/50 (v/v) Protease Inhibitor Cocktail (Sigma). They were homogenized by passing through a 25-G needle for 10 times. Oocyte lysates were incubated by rotating at 4 °C for 1 h. Lysates were centrifuged for 30 min at 10,000 g , and supernatants were collected. The supernatants were mixed with 20 μl anti-FLAG coated beads (EZview Red ANTI-FLAG M2 Affinity Gel from Sigma) and rotated at 4 °C for 2–5 h. The beads were collected and then washed with 400 μl wash solution (lysis solution+500 mM NaCl and 0.5% triton X-100) for three times by rotating at 4 °C for 5 min. Proteins were then eluted with 40 μl 1.5 × SDS loading buffer by incubating at 37 °C for 30 min. Surface protein biotinylation Proteins expressed on Xenopus oocyte plasma membrane were biotinylated and purified with a Pierce Cell Surface Protein Isolation Kit (Pierce) by following a modified protocol. Four to five days after injection, oocytes (30 for each sample) were washed three times with cold OR2 solution (82.4 mM NaCl, 2.5 mM KCl, 1 mM MgCl 2 , 10 mM HEPES, pH 7.6) and placed in six-well plate. Sulpho-NHS-SS-Biotin (2.5 ml 1.2 mg ml −1 ) in ice-cold OR2 was added onto each sample. Sample plate was placed on orbital shaker and gently agitated for 30 min at 4 °C. Quenching solution, 500 μl (from the kit), was added into each sample and incubated for 5 min. Oocytes were then washed with 3 ml Tris-buffered saline for three times and collected into Eppendorf tubes. Lysis buffer, 500 μl (from the kit), and 10 μl protease inhibitor cocktail were added (Sigma) into each sample. Oocytes were homogenized and lysed and the lysates were collected as above. The lysates were mixed with 40 μl NeutrAvidin agrose beads (from the kit) and rotated at 4 °C overnight. Beads were collected by centrifugation and washed for four times. Proteins were eluted by incubating with SDS Blue Loading Buffer with 100 mM DTT at 37 °C for 30 min. SDS–PAGE and western blot SDS–PAGE was run with 10% home-made gel or Invitrogen NuPAGE Novex 4–12% Bis-Tris gel unless otherwise mentioned. Western blot was done with GenScript One Hour Western blot kit with mouse monoclonal anti-HA (Covance), anti-Flag (Sigma) or anti-β actin antibody (GenScript) and Alexa Fluor 680 goat anti-mouse secondary antibody (Invitrogen). Blot membranes were scanned with Odyssey Infrared Imaging System (Li-COR). Band intensity was analysed with the software ImageJ (NIH). Accession codes: The coordinates and structural factors for the TRPP3 coiled-coil domain have been deposited in the Protein Data Bank (PDB) under the accession code 4GIF . How to cite this article: Yu Y. et al . Molecular mechanism of the assembly of an acid-sensing receptor ion channel complex. Nat. Commun. 3:1252 doi: 10.1038/ncomms2257 (2012).